Synthesizing AND gate genetic circuits based on CRISPR-Cas9 for identification of bladder cancer cells The conventional strategy for cancer gene therapy offers limited control of specificity and efficacy. A possible way to overcome these limitations is to construct logic circuits. Here we present modular AND gate circuits based on CRISPR-Cas9 system. The circuits integrate cellular information from two promoters as inputs and activate the output gene only when both inputs are active in the tested cell lines. Using the luciferase reporter as the output gene, we show that the circuit specifically detects bladder cancer cells and significantly enhances luciferase expression in comparison to the human telomerase reverse transcriptase-renilla luciferase construct. We also test the modularity of the design by replacing the output with other cellular functional genes including hBAX , p21 and E-cadherin . The circuits effectively inhibit bladder cancer cell growth, induce apoptosis and decrease cell motility by regulating the corresponding gene. This approach provides a synthetic biology platform for targeting and controlling bladder cancer cells in vitro . Bladder cancer is one of the most common urologic tumours all over the world [1] . Conventional therapies for bladder cancer, such as chemotherapy and radiation, have focused on mass cell killing without specific targeting and often cause side effects and frequent failures [2] . Targeted therapeutic strategy based on human cancer gene therapy is a very promising approach to the treatment of bladder cancer. In this strategy, a vector encoding an apoptotic or cytotoxic gene driven by a cancer-specific promoter is usually used to kill only cancer cells in which the selected promoter is highly active [3] . It requires promoters that are highly active in cancer cells and whose transcriptional activity is undetectable in normal cells. While the selected promoter is abnormally active in cancer cells, it may be also expressed in the normal cells of a different tissue [4] . So one concern associated with this strategy is low specificity. Another concern is that cancer-specific promoters are usually weak promoters that lead to insufficient levels of gene expression [5] . Therefore, new approach for enhancing specificity and availability of cancer gene therapy is required. Although still in its infancy, engineering principles have been applied to programme new biological behaviour, dynamics and logic control in the field of synthetic biology [6] . Various types of nucleic acid- or protein-based Boolean logic gates have been synthesized to control cellular functions [7] . Most of these genetic circuits can work well in prokaryotic or eukaryotic cells and are now being used to build a novel platform for next-generation circuit design. The possibility of constructing logic circuits capable of performing logical functions in mammalian cells was a landmark advance in synthetic biology [8] . Recent works in mammalian synthetic biology have increased the applicability of synthetic logic circuit for human cancer therapy. The design and construction of genetic circuit has thus provided a solution to overcome the limitation of the cancer gene therapy. Bacteria have mechanisms by which they can cleave invading viruses and plasmids, thereby preventing replication of foreign genetic materials. This process is often achieved by CRISPR-associated (Cas) systems. The nuclease Cas9 is the best-characterized member of the Type II CRISPR system and can be used to mediate double strand DNA cleavage and gene knockout in mammalian cells by a sgRNA consisting of a 20-nt guide sequence [9] , [10] , [11] . As the functional complex can only be formed from the combination of the Cas9 and single guide RNA (sgRNA), we proposed that CRISPR-Cas9 system enables the construction of novel logic circuits and opens up new approaches for controlling cellular phenotypes. In this study, we construct the modular AND gate circuits based on CRISPR-Cas9 system by combining the cancer-specific promoter of human telomerase reverse transcriptase (hTERT) gene with the bladder-specific promoter of human uroplakin II gene (hUP II) and test ability of these circuits in selectively indentifying bladder cancer cells. We show that these systems are efficacious in treating human bladder cancer cells. Circuit design and construction We decided to construct a genetic circuit to only operate in bladder cancer cells that behaves as a logical AND gate on two input promoters. The AND gate activates an output that produces a cellular phenotype only when both promoters are capable of driving gene expression in the tested cell lines. This designed circuit is based on the CRISPR/Cas9 system and contains four genes and their promoters, encoded on plasmids ( Fig. 1a ). 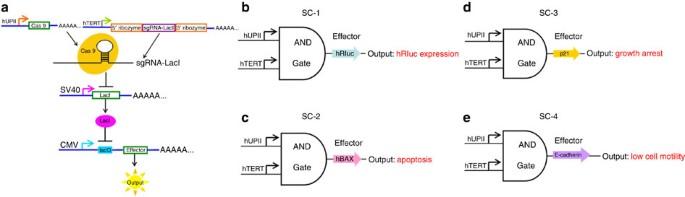Figure 1: Design and construction of the AND gate genetic circuits. (a) The hUP II and hTERT promoters are the inputs to the circuit. The hUP II promoter drives the transcription of Cas9 mRNA and the hTERT promoter is linked to the transcription of sgRNA targeting LacI. The output gene is driven by a LacI-controlled CMV promoter. The effector can be expressed only when both Cas9 protein and sgRNA are presented. (b–e) are schematic representations of the synthetic circuits (SC-1, SC-2, SC-3 and SC-4). The output genes were hRluc, hBAX, p21 and E-cadherin, respectively. Figure 1: Design and construction of the AND gate genetic circuits. ( a ) The hUP II and hTERT promoters are the inputs to the circuit. The hUP II promoter drives the transcription of Cas9 mRNA and the hTERT promoter is linked to the transcription of sgRNA targeting LacI. The output gene is driven by a LacI-controlled CMV promoter. The effector can be expressed only when both Cas9 protein and sgRNA are presented. ( b – e ) are schematic representations of the synthetic circuits (SC-1, SC-2, SC-3 and SC-4). The output genes were hRluc, hBAX, p21 and E-cadherin, respectively. Full size image The first input promoter—hUP II promoter—drives the transcription of mRNA encoding Cas9 protein. The second input promoter—hTERT promoter—drives the transcription of sgRNA-LacI (a sgRNA that targets LacI gene) ( Supplementary Fig. 1 ). The expression of sgRNA under the control of hUP II promoter (a Pol II promoter) is accomplished using two hammerhead ribozymes placed at both ends of sgRNA ( Supplementary Fig. 2 ). When the primary transcript is generated, it undergoes self-catalyzed cleavage to precisely release the designed sgRNA [12] , [13] . To control expression of the output gene—human renilla luciferase (hRluc) ( Fig. 1b )—we used the SV40 constitute promoter to drive the expression of LacI repressor protein. LacI proteins bind to the lac operator sites located adjacent to the strong cytomegalovirus (CMV) promoter of output gene and provide transcriptional repression of output gene. We further confirmed the efficacy ( Supplementary Fig. 3 ) and specificity ( Supplementary Fig. 4 ) of the sgRNA in disrupting LacI. To demonstrate the modularity of the circuit design, we also used hBAX gene ( Fig. 1c ), p21 gene ( Fig. 1d ) and E-cadherin gene ( Fig. 1e ) as the outputs. These genetic circuits can have an output when the Cas9/sgRNA complex binds to the LacI gene through Watson–Crick base pairing and cleaves the DNA sequences. Since the hTERT and hUP II promoters are only both activated at the same time in bladder cancer, we speculated that the output gene in the circuits can be selectively expressed in bladder cancer cells. Detection of bladder cancer cells To investigate the ability of the synthetic circuit (SC-1) in discriminating bladder cancer cells/other cancer cells and normal cells, luciferase assays were performed using four types of bladder cancer cells (T24, 5637, SW-780 and J82), one immortalized cell (293T), three types of other cancer cells (HeLa, A549 and PC-3), two types of normal germ cells (GC-1 and GC-2) and one normal primary fibroblast derived from skin. In theory, the AND gate would only be activated in T24, 5637, SW-780 and J82 cells, all of which have high activities of both hTERT and hUP II promoters. As shown in Fig. 2 , the relative activity of luciferase varied widely among the tested cell lines, but the circuit only demonstrated significant activity in the four bladder cancer cell lines as expected. In contrast, the control Rluc reporter driven by hTERT promoter exhibited significant but weak activity in all cells except in fibroblast. Therefore, the genetic circuit significantly improved output gene expression in all the bladder cancer cell lines examined in comparison to hTERTp-dependent vector. These findings suggest that the constructed circuit behaves as a near-digital AND gate and can be used to specifically identify bladder cancer cells. 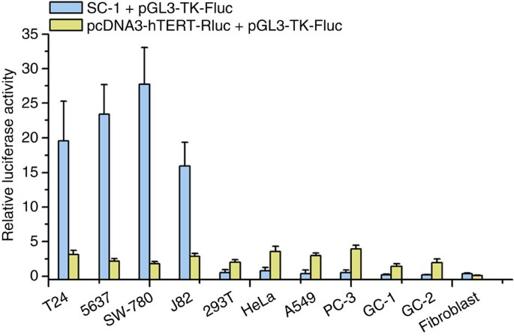Figure 2: Luciferase expression levels of several cell lines transfected with either the synthetic circuit or the hTERT-Rluc vector. All transfections were performed in the presence of PGL3-TK-Fluc vector. Relative luciferase activities are determined as the ratios between Rluc and Fluc values. Each bar shows mean±s.e. Each experiment was performed in triplicate for five independent times. Each error bar indicates the variation between the means of the five independent experiments. Figure 2: Luciferase expression levels of several cell lines transfected with either the synthetic circuit or the hTERT-Rluc vector. All transfections were performed in the presence of PGL3-TK-Fluc vector. Relative luciferase activities are determined as the ratios between Rluc and Fluc values. Each bar shows mean±s.e. Each experiment was performed in triplicate for five independent times. Each error bar indicates the variation between the means of the five independent experiments. Full size image Specific induction of apoptosis of bladder cancer cells Next, we asked whether the circuit (SC-2) can selectively induce apoptosis of bladder cancer cell by regulating expression of human Bax gene, which is a pro-apoptotic gene [14] . As previously reported, Bax protein is a hallmark of cell apoptosis and has the ability to induce apoptosis in a wide variety of cells. The cell-killing ability of the circuit was determined by cell death detection enzyme-linked immunosorbent assay (ELISA) relative to single hTERT promoter construct. As shown in Fig. 3 and Supplementary Fig. 5a , the circuit selectively increased hBAX protein expression and triggered apoptosis in bladder cancer cells without obviously affecting the other cell types. In contrast, the hTERT-hBax construct weakly induced cell apoptosis in all cells except in fibroblast and did not have target specificity for the bladder cancer cells. These results suggest that the constructed circuit is designed to be modular and can be used to specifically and effectively kill bladder cancer cells. 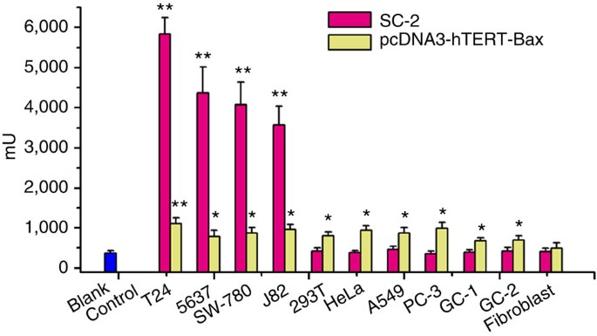Figure 3: Apoptosis levels of several cell lines transfected with either the synthetic circuit or the hTERT-BAX vector. The level of cell apoptosis was calculated using the Cell Death Detection ELISA assay. Results are shown as mean±s.e. The blank control represents cells transfected with the pcDNA3 empty vector. Each experiment was performed in triplicate for five independent times. mU=absorbance [10−3]. *P-value<0.05, and **P-value<0.01, relative to the blank control by two-tailedt-test. Figure 3: Apoptosis levels of several cell lines transfected with either the synthetic circuit or the hTERT-BAX vector. The level of cell apoptosis was calculated using the Cell Death Detection ELISA assay. Results are shown as mean±s.e. The blank control represents cells transfected with the pcDNA3 empty vector. Each experiment was performed in triplicate for five independent times. mU=absorbance [10 −3 ]. * P -value<0.05, and ** P -value<0.01, relative to the blank control by two-tailed t -test. Full size image Specific inhibition of growth of bladder cancer cells We then further determined the modularity of the circuit design and examined whether the circuit (SC-3) can control cell proliferation by regulating expression of p21 gene (also known as cyclin-dependent kinase inhibitor 1A), which is a well-known cell cycle regulator and functions as a molecular break inducing cell growth arrest [15] . Cell proliferation was determined at various time points by CCK-8 assay. Data presented in Fig. 4 and Supplementary Fig. 5b showed that the circuit selectively increased p21 protein expression and strongly suppressed proliferation in bladder cancer cells ( P <0.01 for each cell, analysis of variance (ANOVA)) but not affected non-bladder cells ( P >0.05 for each cell, ANOVA). For hTERT-p21 construct, in contrast, has minimal to moderate effect on the growth of all cells ( P <0.05 for each cell, ANOVA) except normal fibroblast ( P >0.05, ANOVA).These results suggest that the constructed circuit can be used to specifically and strongly inhibit the proliferation of bladder cancer cells. 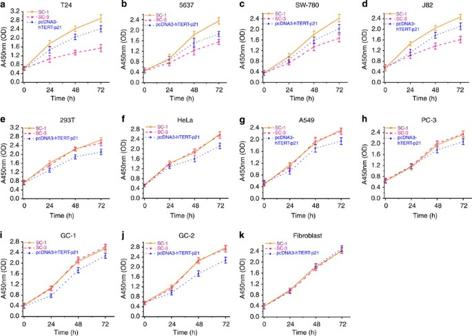Figure 4: Growth curves of several cell lines transfected with either the synthetic circuit or the hTERT-p21 vector. Proliferations of the transfected cells T24 (a), 5637 (b), SW-780 (c), J82 (d), 293T (e), HeLa (f), A549 (g), PC-3 (h), GC-1 (i), GC-2 (j) and fibroblast (k) were measured by CCK-8 assay at different time intervals. The curves of cell proliferation were compared using ANOVA. Result at each time point is shown as mean±s.e. Each experiment was performed in triplicate for five independent times. Each error bar indicates the variation between the means of five independent experiments. Figure 4: Growth curves of several cell lines transfected with either the synthetic circuit or the hTERT-p21 vector. Proliferations of the transfected cells T24 ( a ), 5637 ( b ), SW-780 ( c ), J82 ( d ), 293T ( e ), HeLa ( f ), A549 ( g ), PC-3 ( h ), GC-1 ( i ), GC-2 ( j ) and fibroblast ( k ) were measured by CCK-8 assay at different time intervals. The curves of cell proliferation were compared using ANOVA. Result at each time point is shown as mean±s.e. Each experiment was performed in triplicate for five independent times. Each error bar indicates the variation between the means of five independent experiments. Full size image Specific inhibition of migration of bladder cancer cells Last, the output is swapped from p21 gene to the E-cadherin gene, which is a strong migration suppressor in cells [16] . Loss expression of E-cadherin is thought to contribute to progression in cancer by increasing migration, and/or metastasis. Cell migration was determined by wound-healing assay. Compared with hTERT-E-cadherin construct, the circuit (SC-4) selectively increased E-cadherin protein expression and showed a more robust inhibition of migration in bladder cancer cells ( Fig. 5 and Supplementary Fig. 5c ). In addition, the circuit did not present inhibitory effects on the normal cells and other cancer cells, while the hTERT-E-cadherin construct had small but significant effects on these cells except fibroblast. These data suggest that the constructed circuit can be used to specifically and strongly inhibit the migration of bladder cancer cells. 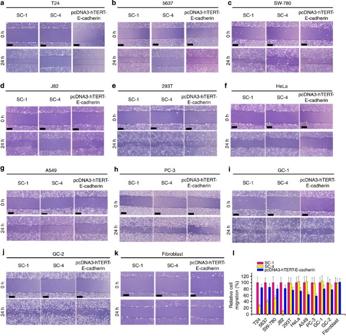Figure 5: Migrations of several cell lines transfected with either the synthetic circuit or the hTERT-E-cadherin vector. Migrations of the transfected cells T24 (a), 5637 (b), SW-780 (c), J82 (d), 293T (e), HeLa (f), A549 (g), PC-3 (h), GC-1 (i), GC-2 (j) and fibroblast (k) were measured by the scratch assay. Data are expressed as mean±s.e. (l). Each experiment was performed in triplicate for five independent times. Each error bar indicates the variation between the means of five independent experiments. Scale bar, 100 μm in each figure. Figure 5: Migrations of several cell lines transfected with either the synthetic circuit or the hTERT-E-cadherin vector. Migrations of the transfected cells T24 ( a ), 5637 ( b ), SW-780 ( c ), J82 ( d ), 293T ( e ), HeLa ( f ), A549 ( g ), PC-3 ( h ), GC-1 ( i ), GC-2 ( j ) and fibroblast ( k ) were measured by the scratch assay. Data are expressed as mean±s.e. ( l ). Each experiment was performed in triplicate for five independent times. Each error bar indicates the variation between the means of five independent experiments. Scale bar, 100 μm in each figure. Full size image A cell is a computing device that mathematically processes multiple input signals to make decisions about their physiological behaviours. The output information of this decision-making process often includes proliferation, migration, division and apoptosis [17] . One goal of synthetic biology is to reconstruct the decision-making circuits by applying engineering principles. Boolean logic gates, capable of performing Boolean logic functions (NOT, AND, OR), are at the core of these biomolecule-based computers [7] . An AND gate is a basic digital logic gate that integrates multiple input signals and has a high output only if all the inputs are high. Different logic AND gates have been built using various biomolecules, such as aptamers [18] , [19] , amber suppressor tRNAs [20] , deoxyribozyme [21] , protein enzyme [22] , repressor proteins [23] and transcriptional effectors [4] , [24] , [25] . It has been proposed that the AND gate can increase the sensing specificity by integrating multiple signals, each of which is too general to identify a specific cellular environment. Genetic circuits based on AND gates can also be used to achieve sensing specificity in cancer therapy. For example, Xie et al . [26] constructed a cell classifier that sensed six different HeLa cell-specific microRNAs and only triggered apoptosis of HeLa cell in all tested cell lines. This work highlights conditional regulation by RNA interference and further strengthens the practicability of SCs in cancer therapy. One obstacle to application of this circuit is that it cannot target other cervical cancer cell lines. In this case it is necessary to construct multiple circuits each capable of identifying one cancer cell line. So such genetic circuits are still to be improved to overcome the limitations. Another system that works on similar principles is the dual-promoter integrator, which integrates information from two cancer-specific promoters to express an anti-cancer output gene [4] . This system can be used to identify and kill cancer cells with a relative high targeting efficacy. However, the synthetic inducible promoter (GAL4) of the output gene used in this work may not always be a strong stable promoter in the tested cell lines. A high level of Gal4 expression can also cause toxicity to normal cells [27] . Moreover, this system is only a one-stage cascade. Addition of more regulatory cascades to the system may further increase steady-state sensitivity and decrease molecular noise [28] . CRISPR/Cas9 system has a notable feature that is desirable for the construction of logic circuits. A sgRNA must combine with Cas9 protein to form an effector complex which guides double-stranded DNA cleavage [11] . As such, the CRISPR/Cas9 system can be incorporated into AND logic gate. However, there is also one drawback to this system. To allow sgRNA to remain in the nucleus, products of sgRNA genes are often transcribed from the Pol III promoters, such as U3 and U6. Unlike Pol II promoters, Pol III promoters are generally constitutive and exhibit no species/tissue specificity. One method to resolve this problem is to generate the RNA molecule with ribozyme sequences at both ends of the sgRNA. The primary transcripts of ribozyme–sgRNA–ribozyme undergo self-catalyzed cleavage and precisely release the sgRNA into nucleus [12] . In this work, we have constructed novel modular AND gate with two-stage cascade based on the CRISPR-cas9 system for targeting human bladder cancer and used the hTERT and hUP II promoters as the two input devices. The hTERT promoter is recognized to be a cancer-specific promoter for various cancers, while it is also activated in the germ line [29] , [30] . The hUPII promoter is a bladder-specific promoter that can only drive gene expression in urothelium cells [31] , [32] . By combining the two promoters into the design, we supposed that the constructed circuits have the ability to selectively indentify bladder cancer cells, in which telomerase and uroplakins are both expressed. To test this hypothesis, we used the luciferase reporter gene as the output of the circuit and tested the relative luciferase activity in exponentially growing normal human cells and cancerous cell lines. The constructed circuit (SC-1) successfully induced bladder cancer-specific gene expression, showing robust luciferase expression in bladder cancer cells, but nearly undetectable luciferase expression in other cell types. In cells with hTERT promoter activity, the circuit induced much higher luciferase expression than single transfection of hTERT-Rluc construct. These results demonstrated that the constructed circuit effectively amplified the response of input promoter to bladder cancer cell endogenous signals and could be a useful detection tool in vitro where the selection of bladder cancer cells is required. Another important feature of the circuit design is modularity. In theory, any output gene can be connected to the AND gate. We placed three functional genes in the end of the circuits and investigated whether the output of the circuits (SC-2, SC-3 and SC-4) could control the behaviours of bladder cancer cells. The results demonstrated that the circuits strongly and specifically inhibited bladder urothelial carcinoma cell growth, induced apoptosis and decreased cell motility by regulating the corresponding gene. In conclusion, this study validated novel genetic circuits that selectively and robustly mediate gene expression in human bladder cancer cells. It would therefore be of great interest to extend these circuits to clinical research when the challenges for in vivo DNA delivery are overcome [33] . Cell lines and cell culture T24, J82, 5637 and SW-780 cells were derived from human bladder cancers and purchased from American Type Culture Collection (ATCC). All cell lines were grown in DMEM medium supplemented with 10% foetal bovine serum (Invitrogen) in the presence of 5% CO 2 . The HEK-293T (embryonic kidney), HeLa (cervical cancer), A549 (lung cancer), PC-3 (prostate cancer), GC-1 (spermatogonium) and GC-2 (spermatogonium) cell lines were also obtained from ATCC and were grown according to the manufacturer’s protocol. Normal human primary fibroblasts derived from the epidermis were kindly provided by Dr T. Chen (Shantou University, Shantou, China) and cultured in defined medium provided by the supplier. SC construction Plasmid hUPII-pSpCas9 (PX165) was constructed by digesting Cbh-3X-FLAG-NLS-SpCas9-NLS (Addgene) with XbaI/AgeI and inserting hUPII promoter fragment into the vector backbone. The hUP II promoter was amplified from human genomic DNA, and the primers used were as follows: forward, 5′- CGTAGCTAGCTGGCAACTTCAAGTGTGGGC -3′ and reverse, 5′- GGCAGGATCCT GGGAGGTGGAATAGGTGCT -3′ [32] . Plasmid RSV-pSpCas9 (PX165) was constructed by digesting Cbh-3X-FLAG-NLS-SpCas9-NLS with XbaI/AgeI and inserting rous sarcoma virus promoter fragment into the vector backbone. The pyrobaculum spherical virus promoter was amplified by PCR from pOPI3CAT (Stratagene). Plasmid hTERT-sgRNA-BAM was constructed by inserting hTERT promoter and ribozyme-flanked sgRNA into pCMVp-NEO-BAM vector (Addgene) at the restriction sites of XbaI/SalI and SalI/BamHI, respectively. The hTERT promoter and the DNA fragment corresponding to designed ribozyme-flanked sgRNA sequences were chemically synthesized. Ribozyme-flanked sgRNAs bearing single mismatches or lacking the complete complementary region were designed and synthesized. To construct the plasmids for expressing these sgRNAs, each of the sequences was individually inserted into hTERT-sgRNA-BAM at the restriction site of SalI/BamHI. Plasmid pRL-SV40-LacI was constructed by inserting LacI gene into pRL-SV40 (Promega) at the restriction site of NheI/XbaI. LacI was amplified by PCR from pCMVLacI (Stratagene). To construct plasmid pcDNA3-LacO-hRluc, the lac operator site and hRluc gene were inserted into pcDNA3 (Addgene) at the restriction sites of Hind III/KpnI and BamHI/EcoRI, respectively. The SV40 intron containing three copies of lac operator site was PCR-amplified from pOPI3CAT. hRluc gene was PCR-amplified from psiCHECK-2 (Promega). To construct plasmids pcDNA3-LacO-hBAX, pcDNA3-LacO-p21 and pcDNA3-LacO-E-cadherin, cDNA sequences for hBAX , p21 and E-cadherin genes were inserted into pcDNA3-LacO-hRluc digested with BamHI/EcoRI, respectively. All three sequences were reverse transcriptase-PCR-amplified from human genomic RNA. Plasmid pcDNA3-hTERT-Bax was created through inserting hTERT promoter and hBax cDNA into pcDNA3 at the restriction sites of NruI/HindIII and BamHI/EcoRI, respectively. Plasmids pcDNA3-hTERT-p21 and pcDNA3-hTERT-E-cadherin were constructed by inserting p21 cDNA and E-cadherin cDNA into pcDNA3-hTERT-Bax digested with BamHI/EcoRI, respectively. Cell transfection For DNA transient transfection experiments, cells were cultured in the plates till they reached 70% confluency and transfected with the mixtures of plasmids using Lipofectamine 2000 (Invitrogen) according to the manufacturer’s protocols. Luciferase assay Luciferase activity was measured in a 1.5-ml Eppendorf tube with the Promega Dual-Luciferases Reporter Assay kit (Promega E1980) according to manufacturer’s protocols at 48 h after transfection. Relative renilla luciferase activity was calculated as value normalized to firefly luciferase activity. The assays were performed in triplicate and the experiments were repeated five times. Western-blot analysis Cells were washed in PBS and lysed in RIPA buffer (50 mM Tris–HCl pH 7.2, 150 mM NaCl, 1% NP40, 0.1% SDS, 0.5% DOC, 1 mM PMSF, 25 mM MgCl 2 and supplemented with a phosphatase inhibitor cocktail). The protein concentration was calculated by using the bicinchoninic acid protein assay. Equal amounts of whole protein extract were electrophoresed on SDS–polyacrylamide gels and then transferred to polyvinylidene difluoride membranes using a semi-dry transfer cell (Bio-Rad Laboratories, Hercules, CA, USA). After blocked with 5% milk, membranes were incubated over night with specific primary antibodies against hBAX (1:1,000; Santa Cruz Biotechnology, Santa Cruz, CA, USA), p21 (1: 200; Santa Cruz Biotechnology), E-cadherin (1:200; Santa Cruz Biotechnology) and GAPDH (1:10,000; Sigma-Aldrich). Then, the blot was incubated with horseradish peroxidase-conjugated secondary antibody (Amersham, Piscataway, NJ, USA) for 1 h at room temperature on a rocking platform. Products were developed on film using Super Signal chemiluminescence reagents (Pierce). Cell apoptosis assay According to the instructions supplied by the manufacturer, the cell apoptosis was determined by quantifying histone-complexed DNA fragments (nucleosomes) in cytoplasm with cell death detection ELISA (Roche Applied Science). The absorbance, which was proportional to the amount of nucleosomes released into the cytoplasm, was measured at 405 nm wavelength by a microplate reader (Bio-Rad). The experiment for each sample was repeated five times independently. Cell proliferation assay Cell proliferation assay was conducted using the Cell Counting Kit-8 (CCK-8) (Beyotime, Shanghai, China) according to the supplier’s instructions. At 0, 24, 48 or 72 h post-transfection, 10 μl of CCK-8 reagent was added to each well of the 96-well plate and the cells were incubated for an hour. Absorbance was read at a wavelength of 450 nm by using a microplate reader. The assays were done five times independently. Cell migration assay Cell migration was determined with the wound-healing assay. Briefly, cells were seeded in 12-well plates at equal density and grown to 80% confluency. Artificial gaps were generated by the sterile pipette tip. Areas of wound were marked and photographed with a digital camera system. Cell migration distance (mm) was calculated by the software programme HMIAS-2000. Each experiment was repeated five times. Statistical analyses Data were expressed as mean±s.e. Significance tests were performed by using SPSS version 17.0 software (SPSS, Chicago, IL, USA).Statistical significance was determined using Student’s t -test or ANOVA and assigned at P <0.05. How to cite this article: Liu, Y. et al . Synthesizing AND gate genetic circuits based on CRISPR-Cas9 for identification of bladder cancer cells. Nat. Commun. 5:5393 doi: 10.1038/ncomms6393 (2014). Accession Codes. cDNA sequence of the ribozyme-flanked sgRNA in plasmid hTERT-sgRNA-BAM have been deposited in the NCBI Genbank Nucleotide database under accession code KM668221 .